PH motifs in PAR1&2endow breast cancer growth Although emerging roles of protease-activated receptor 1&2 (PAR 1&2 ) in cancer are recognized, their underlying signalling events are poorly understood. Here we show signal-binding motifs in PAR 1&2 that are critical for breast cancer growth. This occurs via the association of the pleckstrin homology (PH) domain with Akt/PKB as a key signalling event of PARs. Other PH-domain signal-proteins such as Etk/Bmx and Vav 3 also associate with PAR 1 and PAR 2 through their PH domains. PAR 1 and PAR 2 bind with priority to Etk/Bmx. A point mutation in PAR 2 , H349A, but not in R352A, abrogates PH-protein association and is sufficient to markedly reduce PAR 2 -instigated breast tumour growth in vivo and placental extravillous trophoblast (EVT) invasion in vitro . Similarly, the PAR 1 mutant hPar1-7A, which is unable to bind the PH domain, reduces mammary tumours and EVT invasion, endowing these motifs with physiological significance and underscoring the importance of these previously unknown PAR 1 and PAR 2 PH-domain-binding motifs in both pathological and physiological invasion processes. G protein-coupled receptors (GPCRs) are the largest family in mammalian cells, mediating a plethora of physiological responses [1] , [2] . Despite the fact that GPCRs emerge as oncogenes that regulate cancer-associated signalling networks, their role in tumour biology is not well understood. Indeed, large-scale genome analyses of multiple human tumours have uncovered novel GPCR alterations, as well as aberrant overexpression of GPCRs in cancer [3] , [4] . It is imperative to determine which of the GPCRs are cancer instigators rather than bystanders to enable identification of candidate genes for future targeted personalized medicine. During cancer progression, normal epithelial organization is disrupted and cells are maintained outside their normal niches [5] , [6] . Both soluble and matrix-immobilized proteases are present in the dynamic and flexible microenvironment of a tumour and contribute to the process of cancer advancement [7] . One example is the activation of cell surface protease-activated receptors (PARs). Mammalian PARs are a subgroup of GPCRs that form a four-member family [8] , [9] , [10] , [11] , [12] . PAR 1 and PAR 2 play a central role in epithelial tumour growth in a variety of malignancies [13] , [14] , [15] , [16] . Whereas PAR 2 is not considered a thrombin receptor (unlike PAR 1,3 and 4 ), the PAR 1 -tethered ligand SFLLRN is capable of transactivating PAR 2 (refs 17 , 18 ). Increasing evidence supports the notion that PAR 1 and PAR 2 exist in close proximity and act as one functional unit forming heterodimers [17] , [18] , [19] . Consistently, we have found that PAR 2 plays a dominant role in PAR 1 –PAR 2 -instigated tumour activity [20] . Among the protein modules that drive intermolecular interactions in cellular signalling, the pleckstrin homology (PH) domain is most common. PH domains are mainly recognized by their structural characteristics, and with a seven-stranded β-sandwich and a C-terminal α-helix [21] . While PH domains lack primary sequence similarity, their superfold assembly represents a particularly stable structural scaffold employed in many different functions [22] . Here we describe PH-domain-binding motifs in PAR 1 and PAR 2 C-tails that are necessary for PAR-driven tumour growth and time-limited placental trophoblast invasion. We propose that these PH-domain-binding motifs may serve as an important molecular mechanism within the PAR signalling network and provide a platform for future drug therapy design. PAR 2 associates with Akt/PKB via its PH domain To identify a key signalling partner that plays a role in PAR 2 -driven tumour growth ( Supplementary Fig. 1 ), we analysed the interaction between PAR 2 and Akt/PKB, a serine/threonine protein kinase that plays a pivotal role in tumour cell survival, proliferation and invasiveness [23] , [24] . HEK-293T cells were transiently transfected with hPar2 and cell lysates, before and after SLIGKV-PAR 2 activation, were immunoprecipitated with anti-PAR 2 antibodies and analysed for Akt/PKB co-association. A tight association was observed after 2–10 min of activation, which declined thereafter ( Fig. 1a,b ). This interaction takes place via the binding of PAR 2 C-tail with the PH domain of Akt/PKB, as evaluated by the GST-PAR 2 C-tail pull-down assay ( Fig. 1c ). Akt/PKB also co-associates with PAR 1 via its PH domain ( Supplementary Fig. 2 ). 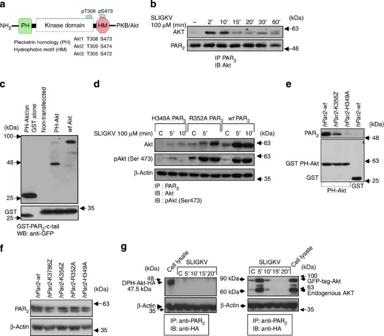Figure 1: Akt/PKB associates with PAR2C-tail via its PH domain. (a) Schematic presentation of Akt/PKB. (b) Immunoprecipitation (IP) analysis of PAR2and Akt/PKB. HEK 293T cells were transfected withwt hPar2. IP was performed following PAR2activation using anti PAR2antibodies and immunoblotting with anti-Akt antibodies. Co-immunoprecipitation (Co-IP) was performed following SLIGKV PAR2activation ofwt hPar2at 2–10 min. (c) GST-PAR2-C-tail bindswtAkt or Akt-PH-domain module alone. HU nearly normal cells (naive cells not expresing endogenous PAR2) were transiently transfected or not with either GFP-wtAkt or GFP-PH-domain alone. Cell lysates were applied to the GST-PAR2C-tail. Specific binding was seen following separation on SDS–PAGE and detection using anti-GFP antibodies. (d) PAR2mutant H349A fails to associate with Akt. HU cells were transiently transfected either withwt hPar2, PAR2mutant R352A or PAR2mutant H349A. Cell lysates were immunoprecipitated following SLIGKV PAR2activation using anti-PAR2antibodies. Detection by western blot analyses of Akt PAR2association was performed using anti-Akt antibodies. Phosphorylation of Akt was detected using anti-phospho Ser473 antibodies. Where indicated, IP detection of PAR2was carried out using anti PAR2SAM11 ab (1 μg per assay) at 1:500 dilution. (e) PAR2mutant H349A fails to associate with GST-Akt-PH domain. Application of HU cells following transient transfection with the indicated constructs (for example,wt hPar2, a shorthPar2C-tail-K356Z and thehPar2mutant H349A) on columns of GST-Akt-PH domain, resulted in effective association as detected by western blot analysis with thewtand PAR2-K356Z constructs. No binding was seen in the presence of the PAR2point mutation H349A. (f) Expression of PAR2constructs. HU cells were transiently transfected with the indicated PAR2constructs. Level of construct expression is detected by Western blot analysis, using anti PAR2antibodies. (g) Delta PH-Akt does not associate with PAR2C-tail. HU cells were transiently transfected withYFP-hPar2construct and either GFP-wt-Akt or myr-Akt delta 4–129 (PH domain) HA-tag. IP was performed following PAR2SLIGKV activation, using anti-PAR2antibodies and immunoblotting with anti-Akt antibodies. While co-association was observed in cells transfected with GFP-wtAkt, in-contrast, no association was seen following SLIGKV PAR2activation in cells transfected with the myr-Akt delta 4–129 (PH-domain) HA-tag plasmid. Control for protein loading is shown by levels of β-actin. Figure 1: Akt/PKB associates with PAR 2 C-tail via its PH domain. ( a ) Schematic presentation of Akt/PKB. ( b ) Immunoprecipitation (IP) analysis of PAR 2 and Akt/PKB. HEK 293T cells were transfected with wt hPar2 . IP was performed following PAR 2 activation using anti PAR 2 antibodies and immunoblotting with anti-Akt antibodies. Co-immunoprecipitation (Co-IP) was performed following SLIGKV PAR 2 activation of wt hPar2 at 2–10 min. ( c ) GST-PAR 2 -C-tail binds wt Akt or Akt-PH-domain module alone. HU nearly normal cells (naive cells not expresing endogenous PAR 2 ) were transiently transfected or not with either GFP- wt Akt or GFP-PH-domain alone. Cell lysates were applied to the GST-PAR 2 C-tail. Specific binding was seen following separation on SDS–PAGE and detection using anti-GFP antibodies. ( d ) PAR 2 mutant H349A fails to associate with Akt. HU cells were transiently transfected either with wt hPar2 , PAR 2 mutant R352A or PAR 2 mutant H349A. Cell lysates were immunoprecipitated following SLIGKV PAR 2 activation using anti-PAR 2 antibodies. Detection by western blot analyses of Akt PAR 2 association was performed using anti-Akt antibodies. Phosphorylation of Akt was detected using anti-phospho Ser473 antibodies. Where indicated, IP detection of PAR 2 was carried out using anti PAR 2 SAM11 ab (1 μg per assay) at 1:500 dilution. ( e ) PAR 2 mutant H349A fails to associate with GST-Akt-PH domain. Application of HU cells following transient transfection with the indicated constructs (for example, wt hPar2 , a short hPar2 C-tail-K356Z and the hPar2 mutant H349A) on columns of GST-Akt-PH domain, resulted in effective association as detected by western blot analysis with the wt and PAR 2 -K356Z constructs. No binding was seen in the presence of the PAR 2 point mutation H349A. ( f ) Expression of PAR 2 constructs. HU cells were transiently transfected with the indicated PAR 2 constructs. Level of construct expression is detected by Western blot analysis, using anti PAR 2 antibodies. ( g ) Delta PH-Akt does not associate with PAR 2 C-tail. HU cells were transiently transfected with YFP - hPar2 construct and either GFP- wt -Akt or myr-Akt delta 4–129 (PH domain) HA-tag. IP was performed following PAR 2 SLIGKV activation, using anti-PAR 2 antibodies and immunoblotting with anti-Akt antibodies. While co-association was observed in cells transfected with GFP- wt Akt, in-contrast, no association was seen following SLIGKV PAR 2 activation in cells transfected with the myr-Akt delta 4–129 (PH-domain) HA-tag plasmid. Control for protein loading is shown by levels of β-actin. Full size image To conclusively identify the critical amino acids involved in this association, point mutations were inserted in the PAR 2 C-tail downstream of the membrane-anchoring site (R352A and H349A, Supplementary Table 1 ). While binding was observed with mutant R352A similar to wt PAR 2 , no association was seen with H349A ( Fig. 1d ). The PAR 2 -bound Akt was functionally active, as demonstrated by high phosphorylation levels of Ser473 ( Fig. 1d ). Importantly, introduction of these mutants did not alter the cell distribution of PAR 2 , as shown by the analysis of the cell surface expression, although truncated hPar2 was expressed to somewhat a lower level ( Supplementary Fig. 3 ). When cell lysates overexpressing either wt hPar2 or a short deleted PAR 2 C-tail construct ( hPar2- K356Z) and mutant hPar2 -H349A were applied to GST-PH-Akt columns, a potent binding association with wt hPar2 and with hPar2 K356Z was obtained. No binding was observed when cell lysates expressing mutant PAR 2 H349A were applied, or when wt hPar2 was applied to GST beads alone ( Fig. 1e ). Levels of the various constructs expression are shown in Fig. 1f . When an Akt construct that was devoid of the PH domain was utilized, no association between PAR 2 and Akt took place ( Fig. 1g ). This provides support for the role of the PH domain of Akt in the binding association between PAR 2 and Akt. Furthermore, the mutant hPar2 -H349A effectively inhibited cell migration and wound closure in a similar way to truncated hPar2 . In contrast, activation of wt hPar2 potently induced migration and closure of the wound by 72 h. SLIGKV activation of mutant hPar2 -R352A induced migration, although at a slower rate compared with wt hPar2 ( Supplementary Fig. 4 ). Other PH-domain signal proteins associate with PAR 1/2 We next examined the possibility that additional signal proteins carrying a PH domain are capable of association with PAR. ExPASy proteomics was used to identify a wide panel of PH-domain-containing proteins. Among others, the signal proteins Etk/Bmx, Akt, Vav, SOS1 and GAB1 were found to carry this domain. We chose to focus on two signalling proteins, Etk/Bmx and Vav 3 . The interaction between PAR 2 and Etk/Bmx, a member of the nonreceptor tyrosine kinase family encoded by the BMX gene [25] , [26] was examined. We previously examined the interaction between Etk/Bmx and PAR 1 (ref. 27 ). Distinct association between PAR 2 and Etk/Bmx was observed at 15–20 min, which declined thereafter ( Fig. 2a–c ). In contrast, no binding was obtained when a truncated form of hPar2 , devoid of the entire cytoplasmic tail, was ectopically expressed in the cells. This association takes place via the binding of the PAR 2 C-tail with the PH domain of Etk/Bmx, as evaluated by the GST-PH-Etk/Bmx pull-down assay ( Fig. 2d ). 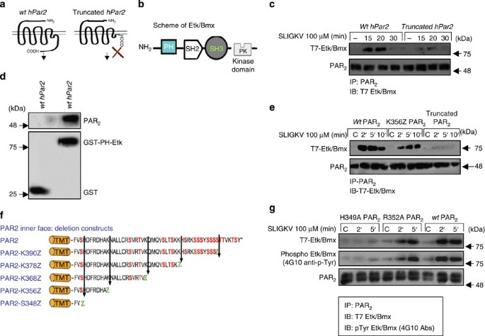Figure 2: Association between PAR2and Etk/Bmx via its PH domain. (a) Schematic presentation ofwtand truncated PAR2. (b) Scheme of Etk/Bmx. (c) HEK293T cells were transfected with T7 Etk/Bmx and eitherwt hPar2or a truncated form ofhPar2plasmids. IP was performed following PAR2activation using anti-PAR2antibodies and immunoblotting with anti-T7 for Etk/Bmx detection (T7 tagged Etk/Bmx) of a Western blot. Effective co-immunoprecipitation was seen following SLIGKV PAR2activation ofwt hPar2but not with a truncated form ofhPar2. (d) PAR2binding to GST-PH-Etk/bmx domain. Cell lysates expressing PAR2were applied on either GST-PH-Etk/Bmx or GST beads alone, specific binding was seen on the GST-PH-Etk/Bmx beads but not on the GST beads, as detected by Western blot analyses. (e) Co-IP betweenwtPAR2and PAR2deleted constructs. HEK293T cells were transiently transfected with the various PAR2constructs. While effective association was seen following SLIGKV PAR2activation in thewtPAR2and the shortest C-tail PAR2K356Z deleted construct, no association was observed in the presence of the truncated form of PAR2, which was devoid of the entire C-tail. (f) Schematic representation of PAR2C-tail deleted constructs. (g) PAR2mutant H349A fails to bind Etk/Bmx. HU cells were transiently transfected with eitherwt hPar2, PAR2mutant R352A, or PAR2mutant H349A. Cell lysates were immunoprecipitated following SLIGKV PAR2activation with anti-PAR2antibodies. Detection for Etk/Bmx PAR2association was carried out by anti-T7 antibodies. Tyr-phosphorylation of bound Etk/Bmx was detected using anti-4G10 antibodies for the detection of phosphotyrosine residues. Levels of PAR2are shown as control. When indicated, detection of PAR2was carried out using either SAM 11ab (Santa Cruz Biotechnology) at1:500 dilution. Figure 2: Association between PAR 2 and Etk/Bmx via its PH domain. ( a ) Schematic presentation of wt and truncated PAR 2 . ( b ) Scheme of Etk/Bmx. ( c ) HEK293T cells were transfected with T7 Etk/Bmx and either wt hPar2 or a truncated form of hPar2 plasmids. IP was performed following PAR 2 activation using anti-PAR 2 antibodies and immunoblotting with anti-T7 for Etk/Bmx detection (T7 tagged Etk/Bmx) of a Western blot. Effective co-immunoprecipitation was seen following SLIGKV PAR 2 activation of wt hPar2 but not with a truncated form of hPar2 . ( d ) PAR 2 binding to GST-PH-Etk/bmx domain. Cell lysates expressing PAR 2 were applied on either GST-PH-Etk/Bmx or GST beads alone, specific binding was seen on the GST-PH-Etk/Bmx beads but not on the GST beads, as detected by Western blot analyses. ( e ) Co-IP between wt PAR 2 and PAR 2 deleted constructs. HEK293T cells were transiently transfected with the various PAR 2 constructs. While effective association was seen following SLIGKV PAR 2 activation in the wt PAR 2 and the shortest C-tail PAR 2 K356Z deleted construct, no association was observed in the presence of the truncated form of PAR 2 , which was devoid of the entire C-tail. ( f ) Schematic representation of PAR 2 C-tail deleted constructs. ( g ) PAR 2 mutant H349A fails to bind Etk/Bmx. HU cells were transiently transfected with either wt hPar2 , PAR 2 mutant R352A, or PAR 2 mutant H349A. Cell lysates were immunoprecipitated following SLIGKV PAR 2 activation with anti-PAR 2 antibodies. Detection for Etk/Bmx PAR 2 association was carried out by anti-T7 antibodies. Tyr-phosphorylation of bound Etk/Bmx was detected using anti-4G10 antibodies for the detection of phosphotyrosine residues. Levels of PAR 2 are shown as control. When indicated, detection of PAR 2 was carried out using either SAM 11ab (Santa Cruz Biotechnology) at1:500 dilution. Full size image We then determined the minimal PH-domain-binding region within the PAR 2 C-tail sequence. For this purpose, we prepared deleted PAR 2 C-tail constructs. Effective co-association with the Etk/Bmx PH domain was observed with the shortest C-tail construct hPar2 -K356Z ( Fig. 2e,f ), and similar with the wt hPar2 construct. Following insertion of mutations into the short K356Z region, we found that in HEK 293T cells overexpressing either R352A or H349A mutants no association was seen with the mutant H349A; however, the R352A mutant did associate with the Etk/Bmx PH domain ( Fig. 2g and supplementary Fig. 5A ). PAR 2 C-tail-bound Etk/Bmx was functionally active, allowing downstream signal association, as demonstrated by induced Tyr-phosphorylation levels ( Fig. 2g ). We therefore conclude that the amino acid histidine at position 349 is critical for the association of PAR 2 with the Etk/Bmx PH domain, as was seen above with Akt/PKB. We observed that, while Akt was abundantly expressed in the cancer cell lines examined, Etk/Bmx expression was restricted to CL1, a prostate cancer cell line ( Fig. 3a ). Lysates of cells expressing endogenous or transfected Etk/Bmx, as well as lysates of cells that do not express Etk/Bmx, were loaded on glutathione S -transferase beads fused to the individual PAR C-tails (either PAR 1 or PAR 2 ) for a pull-down assay. Specific association of Etk/Bmx with both GST-PAR 1 and GST-PAR 2 C-tails was observed ( Fig. 3b ). In contrast, in HCT-116 cells that lack endogenous Etk/Bmx, effective association with Akt was observed for both PAR 1 and PAR 2 C-tails ( Fig. 3b ). 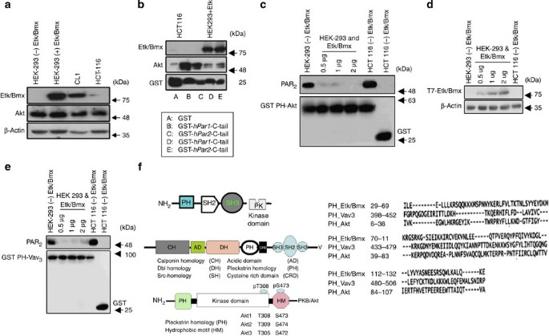Figure 3: PAR1&2C-tails associate with Etk/Bmx or Akt-PH domains. (a) Western blot analysis of Akt and Etk/Bmx in cell lines. Cell lysates of the indicated cell lines were analysed by western blot analysis. Application of anti-Etk/Bmx or anti-Akt antibodies showed that endogenous Etk/Bmx was present only in CL1 cells, an aggressive prostate cancer cell line, or following ectopic overexpression in HEK 293T cells. In contrast, Akt was abundantly present in all the cell lines analysed. (b) PAR1- and PAR2-GST-C-tails associate with Etk/Bmx and Akt. Specific association of the Akt-PH domain was seen in cells that do not express Etk/Bmx (for example, HEK 293T and HCT116 cells). HEK293T cell lysates overexpressingetk/bmxplasmid concentrations (0.5–2 μg) showed no association with the Akt-PH domain. Application of HEK293T cells transfected to overexpress Etk/Bmx showed effective immobilization on both PAR1and PAR2C-tails. Application of HCT116 colon cancer cells that do not express Etk/Bmx showed a marked association with Akt. (c) PAR2binds GST-PH-Akt. Specific association of the Akt-PH domain was seen in cells that do not express Etk/Bmx (for example, HEK 293T and HCT116 cells). HEK293T cell lysates overexpressingetk/bmxplasmid concentrations (0.5–2 μg) showed no association with the Akt-PH domain. (d) Western blot analysis. Levels of T7-Etk/Bmx following increasedetk/bmxplasmid transfection are shown. β-actin was used as a loading control. (e) PAR2binds GST-PH-Vav3. Specific association of the Vav3-PH domain was seen in cells without Etk/Bmx expression (for example, HEK 293T and HCT116 cells). HEK293T cell lysates overexpressingetk/bmxplasmid concentrations (0.5–2 μg) showed no association with the Vav3-PH domain. When indicated, detection of PAR2was carried out using either SAM 11ab (Santa Cruz Biotechnology) at 1:500 dilution. (f) Alignment PH-domain sequences of Etk/Bmx, Vav3and Akt. (d) PAR2binds GST-PH-Vav3.Multiple sequence alignment of PH-Etk/Bmx, PH-Vav3and PH-Akt was performed using T-coffee (available athttp://www.ebi.ac.uk/Tools/msa/tcoffee). Figure 3: PAR 1&2 C-tails associate with Etk/Bmx or Akt-PH domains. ( a ) Western blot analysis of Akt and Etk/Bmx in cell lines. Cell lysates of the indicated cell lines were analysed by western blot analysis. Application of anti-Etk/Bmx or anti-Akt antibodies showed that endogenous Etk/Bmx was present only in CL1 cells, an aggressive prostate cancer cell line, or following ectopic overexpression in HEK 293T cells. In contrast, Akt was abundantly present in all the cell lines analysed. ( b ) PAR 1 - and PAR 2 -GST-C-tails associate with Etk/Bmx and Akt. Specific association of the Akt-PH domain was seen in cells that do not express Etk/Bmx (for example, HEK 293T and HCT116 cells). HEK293T cell lysates overexpressing etk/bmx plasmid concentrations (0.5–2 μg) showed no association with the Akt-PH domain. Application of HEK293T cells transfected to overexpress Etk/Bmx showed effective immobilization on both PAR 1 and PAR 2 C-tails. Application of HCT116 colon cancer cells that do not express Etk/Bmx showed a marked association with Akt. ( c ) PAR 2 binds GST-PH-Akt. Specific association of the Akt-PH domain was seen in cells that do not express Etk/Bmx (for example, HEK 293T and HCT116 cells). HEK293T cell lysates overexpressing etk/bmx plasmid concentrations (0.5–2 μg) showed no association with the Akt-PH domain. ( d ) Western blot analysis. Levels of T7-Etk/Bmx following increased etk/bmx plasmid transfection are shown. β-actin was used as a loading control. ( e ) PAR 2 binds GST-PH-Vav3. Specific association of the Vav 3 -PH domain was seen in cells without Etk/Bmx expression (for example, HEK 293T and HCT116 cells). HEK293T cell lysates overexpressing etk/bmx plasmid concentrations (0.5–2 μg) showed no association with the Vav 3 -PH domain. When indicated, detection of PAR 2 was carried out using either SAM 11ab (Santa Cruz Biotechnology) at 1:500 dilution. ( f ) Alignment PH-domain sequences of Etk/Bmx, Vav 3 and Akt. ( d ) PAR 2 binds GST- PH - Vav3. Multiple sequence alignment of PH-Etk/Bmx, PH-Vav 3 and PH-Akt was performed using T-coffee (available at http://www.ebi.ac.uk/Tools/msa/tcoffee ). Full size image Hierarchy of binding We also examined the priority of binding for Etk/Bmx by adding appropriately modified cell lysates to GST beads fused either to PH-Akt ( Fig. 3c,d ) or to PH-Vav 3 columns ( Fig. 3E ). Vav 3 oncogene, a guanine nucleotide exchange factor (GEF) of the Rho family GTPases, belongs to the Vav protein family [28] , [29] , [30] and is ubiquitously expressed in breast and prostate cancers. Although all Vav family proteins have similar structural features, they display different tissue expression patterns. Vav 1 is primarily expressed in haematopoietic lineages, while Vav 2 is ubiquitously expressed. Vav 3 has a broad but distinct expression profile compared with that of Vav 2 . We showed binding with Vav 3 by a pull-down assay using PH-Vav 3 columns ( Fig. 3e and Supplementary Fig 5B ). 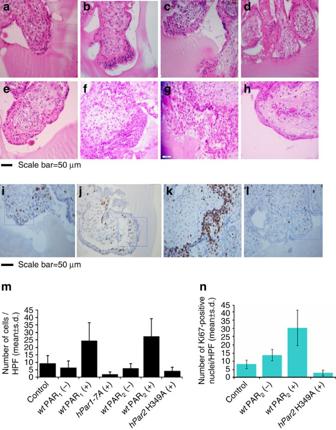Figure 5: Placenta–EVT organ culture invasion. (a–h) Morphology of EVT column growth. Placental explants from the EVT–Matrigel cylinder cast after H&E staining (magnification × 40). Serial 5-μm sections of the Matrigel cylinder were embedded in paraffin blocks prepared for each of the treatment. Images of representative H&E-stained sections at 60 μm depth are presented. (a) Untreated (control), (b)wt hPar1-infected explants, (c) thrombin (1 U ml−1) activation, (d)hPar17A mutant and thrombin activation, (e) control, untreated, (f)wt hPar2, (g)wt hPar2and SLIKGV (100 μM) activation, (h)hPar2mutant H349A and SLIKGV (100 μM) activation. Note the increase in EVT-migrating cells and cell mass at the tip of the villi following either PAR1or PAR2activation. In contrast, a blunt end of the villi without sprouting cells was seen at the villi tip in the presence of mutants following activation treatments. The experiment was terminated 72 h after EVT treatment. Each experiment was performed using three different placentae, in triplicate. (i–l) Immunohistochemical staining of Ki67. Ki67 levels (measure of proliferation) were evaluated in (i) untreated (control), (j) wt hPar2, (k) wt hPar2and SLIKGV (100mM) activation and (l) hPar2mutant H349A and SLIKGV (100mM) activation. (m) Quantification of EVT outgrowth. Cell number was determined at a 60-μm depth of invasion as shown by the histogram mean values. Cells (not the villous compartment) were counted per high-power field (HPF) and expressed as mean±s.e.m.Post hocevaluation of multiple comparisons (ANOVA Tukey HSD) showed aPvalue of 0.0001 within groups. The mean difference was significant at the 0.05 level. ANOVA evaluation was performed with the IBM/SPSS 20.0 software (Chicago, IL, USA). (n) Quantification of Ki67. Histogram of the mean values of Ki67 nuclear staining is shown. Cell nuclei were counted per HPF and expressed as mean±s.e.m.Post hocevaluation of multiple comparisons (ANOVA Tukey HSD) showed aPvalue of 0.0003 within groups. The mean difference was significant at the 0.07 level. ANOVA evaluation was performed with the IBM/SPSS 20.0 software. Before the GST-binding assay, the applied lysates of tumour cell lines were analysed for endogenous expression of either Akt or Etk/Bmx or both. These experiments showed that PAR 1 and PAR 2 have priority for binding with the Etk/Bmx PH domain over Akt or Vav 3 . Only when Etk/Bmx was absent did another PH-domain signal protein such as Akt bind with both PAR 1 and PAR 2 C-tails. PH-Akt/Vav 3 /Etk/Bmx bind to the same site on the PAR 2 C-tail HEK293T cells overexpressing PAR 2 mutants (R352A and H349A) or PAR 2 deletion constructs were added to GST-PH-Etk/Bmx, GST-PH-Akt or GST-PH-Vav 3 . While a specific association was observed with wt hPar2 , hPar2 K368Z and hPar2 K356Z , as well as the mutant R352A, no binding was seen when H349A was added to GST-PH-Etk/Bmx, GST-PH-Akt or GST-PH-Vav 3 ( Fig. 3a–d ). Histidine at position 349 is thus a critical amino acid for PH-signal proteins. Similarly, the same binding region in the PAR 1 C-tail was found for the PH-domain signal proteins tested [27] . Sequence alignment of PH-Etk/Bmx, PH-Vav 3 and PH-Akt showed a high number of different primary sequences ( Fig. 3f ). Characterization of PH-Akt/Etk/Bmx binding There have been a considerable number of reports about the proposed function of Akt PH domain lipid membrane recruitment and AKT activation [31] . AKT is a known phospholipid-binding serine/threonine kinase, and a key component of the phosphoinositide 3-kinase (PI3K) cell survival-signalling pathway that is aberrantly activated in many human cancers [32] . We observed distinct binding of either wt Akt or the GFP-Akt PH domain module alone with the PAR 2 C-tail. In contrast, the Akt PH domain mutant R25C, which has low lipid-binding affinity, failed to associate with PAR 2 ( Fig. 4a ). In addition, the application of LY294002, a PI3K inhibitor, completely abrogated the otherwise potent association between PAR 2 and Akt ( Fig. 4b ). The involvement of phosphatidylinositol (3,4,5)-trisphosphate (PtdIns(3,4,5)P3; PIP3) in the PAR 2 –Akt association is supported by the potent inhibition of PAR 2 -Akt binding in the presence of Ins (1,3,4,5) P4 (IP4) ( Supplementary Fig. 6 ). We conclude that the Akt–PAR 2 association involves membrane anchoring via the PH domain. On the other hand, both the PH domain mutant R28C of the Etk/Bmx PH domain, which is incapable of lipid binding, and the GFP-Etk/Bmx PH domain module alone, exhibited potent binding with PAR 2 C-tail ( Fig. 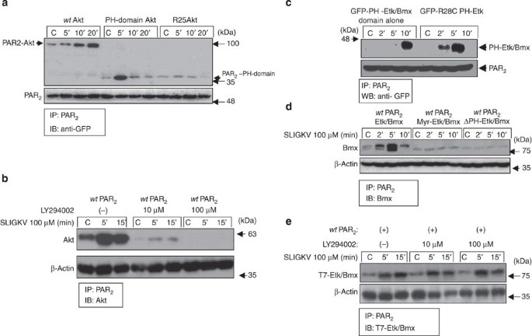4c ). Figure 4: Mechanisms of Akt-PH and Etk/Bmx-PH domain binding to PAR2. (a) PH-Akt module binds PAR2-C-tail but not mutant R25C. HU cells were transiently transfected withhPar2construct and either with GFP-wt-Akt, GFP-PH-Akt domain alone or GFP-R25C. Immunoprecipitation of cell lysates following PAR2activation was carried out using anti-PAR2antibodies. Detection of eitherwtAkt or Akt-PH domain alone associated with PAR2was performed with anti-GFP. WhilewtGFP-Akt and GFP-PH domain alone were shown to bind PAR2, no binding was obtained when the mutant R25C of low lipid-binding-affinity was present. (b) PI3K inhibitor (LY 294002) inhibits binding of Akt to PAR2. Treatment of HU cells with increasing concentrations of LY294002 following transient transfection withhPar2and SLIGKV activation was performed. Cell lysates were immunoprecipitated with anti-PAR2antibodies, and anti-Akt was used to assess the association of Akt with the PAR2C-tail. A potent inhibition of Akt-PAR2association was observed in the presence of LY294002. (c) GFP-PH-Etk/Bmx module and mutant R28C bind PAR2. HU cells were transiently transfected withhPar2construct and with either GFP-PH-Etk/Bmx domain alone or GFP-R28C Etk/Bmx mutant with low lipid-binding affinity. Immunoprecipitation of cell lysates following PAR2activation was performed using anti-PAR2antibodies. Anti-GFP was used to detect the intact Etk/Bmx-PH domain alone associated with PAR2and the mutant R28C. Both constructs bind PAR2potently. (d) Co-IP betweenwtand Etk/Bmx modulation constructs. Co-IP analyses performed utilizing HU cells transiently transfected with eitherwt hPar2,wtEtk/Bmx, Myr-dPH construct or TH-SH2-SH3-KD. No association between Etk/Bmx and PAR2was observed either with Myr-dPH constructs or TH-SH2-SH3-KD construct deleted for the PH domain. In comparison, effective association was obtained withwtEtk/Bmx. (e) LY294002 does not inhibit association of Etk/Bmx with PAR2. Treatment of HU cells with increasing concentrations of LY294002 following transient transfection with both T7-etk/bmxandhPar2and SLIGKV activation was performed. Cell lysates were immunoprecipitated with anti-PAR2antibodies and Etk/Bmx- PAR2association byanti-T7. Figure 4: Mechanisms of Akt-PH and Etk/Bmx-PH domain binding to PAR 2 . ( a ) PH-Akt module binds PAR 2 -C-tail but not mutant R25C. HU cells were transiently transfected with hPar2 construct and either with GFP- wt -Akt, GFP-PH-Akt domain alone or GFP-R25C. Immunoprecipitation of cell lysates following PAR 2 activation was carried out using anti-PAR 2 antibodies. Detection of either wt Akt or Akt-PH domain alone associated with PAR 2 was performed with anti-GFP. While wt GFP-Akt and GFP-PH domain alone were shown to bind PAR 2 , no binding was obtained when the mutant R25C of low lipid-binding-affinity was present. ( b ) PI3K inhibitor (LY 294002) inhibits binding of Akt to PAR 2 . Treatment of HU cells with increasing concentrations of LY294002 following transient transfection with hPar2 and SLIGKV activation was performed. Cell lysates were immunoprecipitated with anti-PAR 2 antibodies, and anti-Akt was used to assess the association of Akt with the PAR 2 C-tail. A potent inhibition of Akt-PAR 2 association was observed in the presence of LY294002. ( c ) GFP-PH-Etk/Bmx module and mutant R28C bind PAR 2 . HU cells were transiently transfected with hPar2 construct and with either GFP-PH-Etk/Bmx domain alone or GFP-R28C Etk/Bmx mutant with low lipid-binding affinity. Immunoprecipitation of cell lysates following PAR 2 activation was performed using anti-PAR 2 antibodies. Anti-GFP was used to detect the intact Etk/Bmx-PH domain alone associated with PAR 2 and the mutant R28C. Both constructs bind PAR 2 potently. ( d ) Co-IP between wt and Etk/Bmx modulation constructs. Co-IP analyses performed utilizing HU cells transiently transfected with either wt hPar2 , wt Etk/Bmx, Myr-dPH construct or TH-SH2-SH3-KD. No association between Etk/Bmx and PAR 2 was observed either with Myr-dPH constructs or TH-SH2-SH3-KD construct deleted for the PH domain. In comparison, effective association was obtained with wt Etk/Bmx. ( e ) LY294002 does not inhibit association of Etk/Bmx with PAR 2 . Treatment of HU cells with increasing concentrations of LY294002 following transient transfection with both T7- etk/bmx and hPar2 and SLIGKV activation was performed. Cell lysates were immunoprecipitated with anti-PAR 2 antibodies and Etk/Bmx- PAR 2 association byanti-T7. Full size image To better characterize the nature of binding between PAR 2 and the Etk/Bmx PH domain, analyses of additional Etk/Bmx constructs were carried out. These constructs were an Etk/Bmx construct whose PH domain was replaced by a myristoyl group attached to the N-terminal portion, Myr-dPH, and a construct depleted of the PH-domain containing the kinase domain, SH3, and SH2 domains, TH-SH2-SH3-KD (refs 33 , 34 ). On SLIGKV activation of PAR 2 , no association between Myr-dPH Etk/Bmx and PAR 2 was observed ( Fig. 4d ). Similarly, no interaction was seen when a deleted PH domain TH-SH2-SH3-KD construct was used ( Fig. 4d ). Accordingly, the presence of LY294002 PI3K inhibitor did not abrogate the association between PAR 2 and Etk/Bmx ( Fig. 4e ). Hence, the Etk/Bmx PH domain association is completely lipid-independent and binds via a protein–protein interaction. This stands in contrast to Akt PH domain association with PAR 2 C-tail, which is membrane lipid-dependent. PAR 2 PH-domain-binding site is critical for EVT invasion Establishment of human pregnancy involves the well-orchestrated invasion to the uterus wall of specialized cells termed extravillous trophoblasts (EVT). We have utilized an in vitro model based on isolation of villi from early gestation human placentae plated on Matrigel [20] , [35] , [36] , [37] . Placental specimens were harvested at the end of the first trimester (10–12 weeks) and those expressing little or no endogenous PAR 1 and PAR 2 were selected. These cultures were transfected with lentiviral wt hPar1 , viral hPar1-7 A mutant, wt hPar2 , or hPar2 mutant H349A, and were activated by their respective ligands. The impact of PAR 1 or PAR 2 activation on wt and mutant forms was evaluated by comparing the depth of invasion. EVT invasion into the Matrigel reached a maximal invasion depth of 100 μm, as evaluated by 5-μm serial sections of the Matrigel cast. Histological analyses of haematoxylin and eosin (H&E) staining are shown in Fig. 5a–h . Significant inhibition in EVT cell invasion was seen in the presence of the mutants that are incapable of association with PH-domain signal protein/s (activated hPar1- 7A or hPar2 H349A, Fig. 5a , lanes d and h, respectively), and before activation ( Fig. 5a , b and e). In contrast, a high level of invasion was observed following either TFLLRN PAR 1 or SLIGKV PAR 2 activation, with invasion reaching up to 100 μm. Highly proliferative EVT cells at the tip of the villi recapitulate outgrowth and depth of invasion. Nuclear staining of ki67 demonstrates the extent of proliferating cells following wt hPar2 and the mutant forms following activation ( Fig. 5i–l ). The number of cells per high-power field for each treatment was evaluated at an equal level of invasion (60 μm), as shown in the representative histogram ( Fig. 5m–n ). Figure 5: Placenta–EVT organ culture invasion. ( a – h ) Morphology of EVT column growth. Placental explants from the EVT–Matrigel cylinder cast after H&E staining (magnification × 40). Serial 5-μm sections of the Matrigel cylinder were embedded in paraffin blocks prepared for each of the treatment. Images of representative H&E-stained sections at 60 μm depth are presented. ( a ) Untreated (control), ( b ) wt hPar1 -infected explants, ( c ) thrombin (1 U ml −1 ) activation, ( d ) hPar1 7A mutant and thrombin activation, ( e ) control, untreated, ( f ) wt hPar2 , ( g ) wt hPar2 and SLIKGV (100 μM) activation, ( h ) hPar2 mutant H349A and SLIKGV (100 μM) activation. Note the increase in EVT-migrating cells and cell mass at the tip of the villi following either PAR 1 or PAR 2 activation. In contrast, a blunt end of the villi without sprouting cells was seen at the villi tip in the presence of mutants following activation treatments. The experiment was terminated 72 h after EVT treatment. Each experiment was performed using three different placentae, in triplicate. ( i – l ) Immunohistochemical staining of Ki67. Ki67 levels (measure of proliferation) were evaluated in ( i ) untreated (control), ( j ) wt hPar 2 , ( k ) wt hPar 2 and SLIKGV (100mM) activation and ( l ) hPar 2 mutant H349A and SLIKGV (100mM) activation. ( m ) Quantification of EVT outgrowth. Cell number was determined at a 60-μm depth of invasion as shown by the histogram mean values. Cells (not the villous compartment) were counted per high-power field (HPF) and expressed as mean±s.e.m. Post hoc evaluation of multiple comparisons (ANOVA Tukey HSD) showed a P value of 0.0001 within groups. The mean difference was significant at the 0.05 level. ANOVA evaluation was performed with the IBM/SPSS 20.0 software (Chicago, IL, USA). ( n ) Quantification of Ki67. Histogram of the mean values of Ki67 nuclear staining is shown. Cell nuclei were counted per HPF and expressed as mean±s.e.m. Post hoc evaluation of multiple comparisons (ANOVA Tukey HSD) showed a P value of 0.0003 within groups. The mean difference was significant at the 0.07 level. ANOVA evaluation was performed with the IBM/SPSS 20.0 software. Full size image PAR 2 Histidine349 is critical for tumour growth in vivo The physiological significance of the PAR 2 PH domain motif is also demonstrated using a xenograft model of tumour growth ( Fig. 6a–c ). We generated stable clones of a nearly normal fibrocystic cell line HU that lacked expression of endogenous PAR 2 but expressed a luciferase construct and one of the following plasmids: wt PAR 2 , a truncated PAR 2 , and PAR 2 mutants; R352A; or mutant R349A ( Fig. 6d ). The stable clones were inoculated subcutaneously into nude mice and were analysed for tumour growth. While large and vascularized tumours developed in mice inoculated with wt PAR 2 , no to minimal change in tumour size was seen in mutant R352A, and markedly smaller tumours were observed with the PAR 2 mutant H349A, compared with PAR 2 -truncated clones ( Fig. 6a–c ). As mentioned above, the PAR 2 R352A mutant did not abrogate PAR 2 association with Etk/Bmx, Akt and the PH domain of Vav 3 ( Fig. 3c,d ). In contrast, mutant H349A effectively abrogated the PAR 2 association with all PH-domain signal proteins tested; hence, His (H) at position 349 is a critical amino acid for binding to all proposed downstream PH-domain signal proteins. Approximately 20-fold larger tumours were observed in mice inoculated with wt hPar2 cells (825 mm 3 ; P <0.0007) as compared with those in mice inoculated with control cells (40 mm 3 ). In a Matrigel invasion assay, wt PAR 2 consistently elicited a significantly higher level of HU cell invasion following PAR 2 activation. In contrast, in the presence of PAR 2 H349A, no Matrigel invasion was observed, comparable to levels in control mice, regardless of SLIGKV activation ( Supplementary Fig. 7 ). Likewise, when a mutated form of hPar1 ( hPar1-7A ) incapable of associating with the PH domain of Etk/Bmx ( hPar1-7A ) was analysed in a murine xenograft mammary model in vivo , a dramatic reduction in the otherwise large tumours was observed ( Supplementary Figs 8 and 9 ). 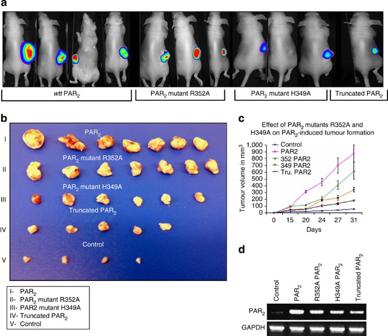Figure 6: PAR2PH-domain-binding sequence is essential for tumour growthin vivo. Stable clones of HU cells were prepared expressing luciferase and eitherwt hPar2,or a truncatedhPar2(devoid of the cytoplasmic tail), or PAR2mutant R352A, or PAR2mutant H349A. The various clones (3 × 106cells) were inoculated subcutaneously in nude mice. (a) Representative bioluminescence images. Levels of tumour luciferase following various cell-clone inoculation treatments. (b) Tumour morphological appearance. At the end of the experiment (for example, within 31 days; I–V), mice were terminated and the tumours (I–V) were excised, measured and weighed. (c) Measurements of tumour volume. Tumours were weighed and measured for size at the indicated time points and tumour volume (mm3) was calculated. Error bars show s.d.; *P<0.005. Data shown are representative of three independent experiments. (d) Levelswtand modified PAR2in the stable clones. Stable clones expressing the varioushPar2constructs, eitherwt hPar2or truncatedhPar2, hPar2mutant R352A or mutant H349A, are shown using PCR. GAPDH levels were used as the control housekeeping gene. Figure 6: PAR 2 PH-domain-binding sequence is essential for tumour growth in vivo. Stable clones of HU cells were prepared expressing luciferase and either wt hPar2, or a truncated hPar2 (devoid of the cytoplasmic tail), or PAR 2 mutant R352A, or PAR 2 mutant H349A. The various clones (3 × 10 6 cells) were inoculated subcutaneously in nude mice. ( a ) Representative bioluminescence images. Levels of tumour luciferase following various cell-clone inoculation treatments. ( b ) Tumour morphological appearance. At the end of the experiment (for example, within 31 days; I–V), mice were terminated and the tumours (I–V) were excised, measured and weighed. ( c ) Measurements of tumour volume. Tumours were weighed and measured for size at the indicated time points and tumour volume (mm 3 ) was calculated. Error bars show s.d. ; * P <0.005. Data shown are representative of three independent experiments. ( d ) Levels wt and modified PAR 2 in the stable clones. Stable clones expressing the various hPar2 constructs, either wt hPar2 or truncated hPar2, hPar2 mutant R352A or mutant H349A, are shown using PCR. GAPDH levels were used as the control housekeeping gene. Full size image It is interesting to note that neutrophil elastase (NE) is incapable of inducing the PAR 2 -PH-Etk/Bmx association ( Supplementary Fig. 10 ), while association of PAR 1 to either PH-Etk/Bmx or PH-Akt is elicited by NE ( Supplementary Fig. 11 ). PH domains are conserved protein motifs present in diverse signal-transducing proteins. They are known to be versatile modules in protein–protein interaction platforms in a plethora of physiological events [38] , [39] . We describe binding motifs capable of selective association with PH domains of Etk/Bmx, AKT and Vav 3 in the C-tails of mammalian PAR 1 and PAR 2 . These binding motifs are necessary for tumour development as well as physiological placental EVT–uterus interactions. Mutations inserted to the PAR 1 PH domain ( Supplementary Figs 7 and 8 ) and point mutation at H349A in PAR 2 markedly attenuated xenograft tumour growth in a murine model of cell migration ( Supplementary Fig. 4 ) and of placental–trophoblast time-limited invasion. Despite the fact that sequence identity between PH domains is limited, their tertiary structures are strikingly similar. Although little is known about the molecular basis of PH-domain function, several lines of evidence indicate that these domains are critical for receptor activity. For example, coupling of insulin receptor and insulin receptor substrate, IRS-1, depends in part on the IRS-1 PH domain [40] , [41] . The PH domain of β-adrenergic receptor kinase is required for its interaction with the βγ-subunits of heterotrimeric G-proteins [42] . Whereas many studies have addressed PH-domain-phospholipid-binding properties, protein–protein interactions are only now being investigated [43] . The PH domain of oncogenic Dbl mediates targeting to the cytoskeletal matrix and was found to be necessary for oncogenic transformation [44] . The PH domains in guanine nucleotide-binding proteins are essential for C-terminal association with the Dbl homology (DH) RhoGEF catalyst. Furthermore, phosphoinositol-lipid-binding PH sites are effective modules for both small guanine nucleotide-binding proteins [45] , [46] and Gα-subunits [47] . Thus, both lipid-binding capabilities and protein–protein interactions play roles in PH-domain module interactions. AKT activation is driven by binding of the PH domain to PIP3 or PIP2 for membrane localization, followed by the phosphorylation of serine 473 and threonine 308 (ref. 48 ). In addition, the PH domain plays a critical regulatory role in AKT function, and mutations disrupting the PH-domain function are apparently important in physiological and disease processes. For example, in a drosophila model, PIP3 levels are lethal when PTEN is lacking. Rescue survival is possible only if the drosophila AKT PH domain is inactive and incapable of binding lipid [49] . This indicates that AKT is a critical target, activated by increased PIP3, for a second lipid messenger pathway. A point mutation introduced into the PH-domain lipid-binding pocket of AKT1, whereby arginine is replaced by cysteine at amino acid 25 (AKT1R25C), results in low-affinity AKT-phospholipid binding, with both inhibited recruitment of AKT to the membrane and association with PAR 2 (ref. 50 ). In another lipid-binding pocket mutation of the AKT–PH domain, E17K alters interactions of the pocket and activates AKT1 by means of pathological localization to the plasma membrane [51] . This mechanism suggests a direct role for AKT1 in human cancer and adds to the known genetic alterations that promote oncogenesis through the phosphatidylinositol-3-OH kinase/AKT pathway. Our data demonstrate that PAR 1 and PAR 2 harness the AKT pathway via binding to their PH domains, thus enabling their downstream network signalling. It is well established that PIP3 functions to activate AKT via binding to the PH-domain-mediating translocation to the plasma membrane for the appropriate downstream signalling. Ins (1,4,5)P3 (IP3) however can be converted to IP4 by a family of inositol trisphosphate kinases. Once generated, IP4 can act as a soluble analogue of PIP3 and thereby negatively regulates PIP3 AKT-PH signalling. Indeed, our data show that potent inhibition of the association between PAR 2 and PH-Akt that requires PIP3 is observed in the presence of increased IP4 concentrations ( Supplementary Fig. 6 ). This regulation is similar to that of other diverse critical decision processes downstream of many receptors. Specific examples are the negative regulation of neutrophil signalling and chemotaxis [52] , neutrophil survival and bacteria killing by neutrophils, of overall importance for neutrophil function and innate immunity [53] . Naturally occurring mutations in the PH domain of Bruton’s tyrosine kinase interfere with phosphoinositide-binding properties and with X-linked agammaglobulinaemia in humans and X-linked immunodeficiency in mice [54] . Here we show that, in contrast to Akt PH domain lipid-binding dependency, the PH domain of Etk/Bmx binds PAR 2 in a phospholipid-independent manner. This is based on the strong PAR 2 -Etk/Bmx association with the mutant that is incapable of binding lipids, and on the lack of association of modified Etk/Bmx constructs, in which the PH domain was replaced with a myristoyl group or with a depleted PH domain construct. This finding is in line with other Etk/Bmx protein–protein interactions, such as binding to the FAK-FERM domain [55] . It was similarly demonstrated that the PH domain of an Etk/Bmx lipid-binding-deficient mutant retained potent FAK-binding capability, indicating that the regulation and association of Etk/Bmx by FAK is independent of lipid-binding activity of the PH domain. Vav 3 proto-oncogene is a member of Vav belonging to the Dbl family of GEF for the Rho family of GTP-binding proteins. The characteristic structural domains of the family include an N-terminal calponin homology domain, an acidic region, a DH domain and a PH domain, among others. Generally, in these protein families the PH domain is located at the C-terminal DH helix and contributes to the support of GEF activity [56] , [57] . It is possible, but remains to be shown, that the preference for Etk/Bmx association with PARs over the Akt or Vav 3 PH domain is due to direct protein–protein interactions, independent of lipid involvement, although the nature of the PH-Vav 3 interaction remains to be fully determined. Overall, regardless of unusually different primary sequences, PH domains share a conserved fold made up of a b-barrel composed of two roughly perpendicular, antiparallel beta-sheets and a C-terminal alpha amphipathic helix. On binding to phosphatidylinositol lipids, a key membrane constituent, PH domains act in the recruiting of proteins to the cell membrane. A large number of PH domains, however, have poor affinity for phosphoinositides and, in fact, function as protein-binding domains. Hence, PH domains are involved in the formation of signalling complexes involved in cell fate decisions and require precise temporal and spatial control. They may employ multiple biologically optimized interaction surfaces that together form a cooperative signalling device. As for the hierarchy, the best interaction between PAR 1&2 C-tails and PH domains takes place via protein–protein interaction, as with Etk/Bmx. However, since these interactions are of high importance, a back-up system is also available in cases when Etk/Bmx is absent in a specific physiological context, for example, in a PH-Akt association. In summary, PH motifs for binding associations, either with lipids that are located within cellular membranes, or via protein–protein interactions, exemplify how the interplay between distinct motifs in a signal protein not only support transmission of a biochemical signal but also ensure a robust response to developmental cues, at precisely the right time, and with sufficient specificity to safeguard against premature and hence disastrous induction of cell fate change. Biased signalling at GPCRs has redefined classical concepts in receptor pharmacology, not only highlighting the depth of signalling diversity within the GPCR system but also offering possibilities for more effective therapeutics [58] , [59] . We have now explored NE’s role in determining the consequences of PH-Etk/Bmx-binding association with either PAR 1 or PAR 2 . NE did not elicit the association of either of the PH-domain signal proteins analysed, Etk/BMX and Akt, with PAR 2 ( Supplementary Fig. 10 ). In contrast, NE was capable of eliciting PAR 1 association with both PH-Etk/BMX and PH-Akt ( Supplementary Fig. 11 ). This dichotomy can be explained by the NE cleavage site locations on PAR 2 versus PAR 1 . While the main digestion site of the PAR 2 N-terminal extracellular domain is rather far downstream from the canonical trypsin cleavage site and is allocated to residues F (67) and (68) SAS, NE cleaves PAR 1 only four residues after the classical thrombin-cleaving site (41) R/ (42) SFLLRN, after L residue L (45) /R (46) NPNDKY. Our NE data are still preliminary and were not the focus of the current study. However, it appears that, at least with regard to PAR 1 , rather than disarming its function, the induced PH-Etk/BMx and/or PH-Akt association joins the MAPK activation previously demonstrated for NE but not for other neutrophil proteinases (for example, proteinase-3 and cathepsin G) [60] , [61] , [62] . The possibility that endogenous NE may be capable of instigating a key PAR 1 signalling event, albeit to a diminished extent compared with classical activation, may be important. This proteinase is abundant in the surroundings of a tumour, providing support to the axis in terms of inflammation-induced tumour development. Other PAR 2 C-tail sequences have been described as having an impact on PAR 2 -induced cellular functions. A sequence region immediately downstream to the PH-domain-binding motif, allocated to residues 356–363, was found to affect PAR 2 -induced InsP 3 accumulation, Ca ++ mobilization and PYK activation. However, the role of this sequence is not clear. It was suggested that perhaps it has to do with the deletion of a palmitoylation site that is usually recognized by a cystein flanked by basic amino-acid residues, as is the case with residues 356–363 (ref. 63 ). In addition, Vogel’s group has demonstrated crosstalk and physical interaction between PAR 2 and TLR4, a member of the Toll-like receptor (TLR) family [64] . TLRs serve as important guards of the innate immune response through their ability to sense conserved pathogen-associated molecular patterns. The C-tail region sequence of PAR 2 , where the physical interaction with TLR4 takes place, is currently unknown and remains to be fully elucidated. Whether PAR 2 PH-domain is critically involved in these interactions is an open question. The three intracellular loops designated C1, C2 and C3 along with the C-tail, termed C4, are critical for class A GPCR signalling, and are recapitulated by interaction with the heterotrimeric G-proteins (for example, α, β and γ subunits) [65] . In general, C1 is the shortest in length, with relatively conserved length between family members, whereas the highest degree of variability is found in C3 and C4 (ref. 66 ). Ligand binding to GPCRs mediates a large conformational change most notably among others, in C2 and C3, which in turn promote activation of G-proteins by exchange of GDP for GTP on the Gα subunit [67] . An array of components composed of a lipid moiety (for example, palmitate, myristate and lithocholic acid) attached to a peptide that corresponds to an amino-acid segment of the cytoplasmic loops (C1, C2 or C3) or the C-terminal tail have shown however to affect all three intracellular loops and also C4, suggesting that all intracellular domains may be important for signal transduction. Within the C-terminal domain is the highly conserved eighth helix (H8) previously identified in rhodopsin [65] and other Class A receptors, including PAR 1 (ref. 68 ) and PAR 2 (ref. 69 ). H8 is anchored to the membrane by palmitoylation of C-terminal cysteine residues. In fact, the PAR 1 PH domain is localized within the H8 loop and was found to be confined to this region. Similarly, palmitoylation of PAR 2 is necessary for post-translational modification and is required for efficient cell surface expression and desensitization of PAR 2 . Our data demonstrate for the first time that PH-domain-binding motifs in the PAR 1 and PAR 2 C-tails are critical signal-initiating sites. These findings define a molecular path in PAR-induced signalling networks. These sites are potential targets for future drug design. It is possible that other cancer ‘driver’ GPCRs harbour PH-domain-binding motifs within their C-tails, which would contribute a more general significance to these sites. This possibility needs to be fully explored. Cell culture HEK-293T, MCF-7, HCT-116 and CL-1 cells (obtained from the American Type Culture Collection) were grown in DMEM. HU breast epithelial cells were generated by the late Dr Aviva Horowitz (member and friend of the Sharett Institute of Oncology, Hadassah-Hebrew University Medical Center, Jerusalem, Israel). The cells were grown in RPMI, supplemented with 1 mM L-glutamine, 50 μg ml −1 streptomycin, 50 U ml −1 penicillin (GIBCO-BRL, Gaithersburg, MD, USA) and 10% fetal calf serum (Biological Industries, Beit Haemek, Israel). Cells were maintained in a humidified incubator with 8% CO 2 at 37 °C. Plasmids and transfection A cDNA encoding wild-type human Par2 was kindly provided by Professor Morley D. Hollenberg (Faculty of Medicine, University of Calgary, Alberta, Canada). Etk/Bmx viral vector and GST-PH-Etk/Bmx constructs were kindly provided by Dr Yun Qiu (Departments of Pharmacology and Experimental Therapeutics, University of Maryland School of Medicine, Baltimore, MD, USA). The GST-PH-Akt construct was kindly provided by Dr Brian A. Hemmings (Friedrich Miescher Institute, Basel, Switzerland). The GST-PH-Vav 3 construct was kindly provided by Dr Shan Lu (University of Cincinnati College of Medicine, Cincinnati, OH, USA). Cells were grown to 70–80% confluency and transfected with 0.1–3.5 μg of plasmid DNA in TransIT LT1 transfection reagent (Mirus Bio LLC, Madison, WI, USA) according to the manufacturer’s instructions. Cells were collected 48 h after transfection and protein lysates/RNA were purified. MCF-7, HU or HEK 293T were grown to 70–80% confluency and transfected with 1–2 μg of either wt human hPar1 or hPar2 or truncated hPar2 (devoid of the cytoplasmic tail) cDNA, or with several hPar2 -deleted constructs, or with a control pcDNA3 vector (Invitrogen, Carlsbad, CA, USA) using TransIT LT1 transfection reagent (Mirus Bio LLC). Transfected cells were selected with G418 (800 μg ml −1 ) to obtain stable populations of cells expressing hPar1 and hPar2 , or hPar1 and truncated hPar2 . PAR 1 and PAR 2 activation Thrombin receptor-activating peptides TFLLRNPNDK for activation of PAR 1 and SLIGKV for PAR 2 were from GenScript (Piscataway, NJ, USA). Thrombin was obtained from OMRIX Bio Pharmaceutical (Ramat Gan, Israel). Gateway cloning The wt hPar1 (or) hPar1 7A, wt hPar2 and mutant hPar2 H349A-coding sequence was cloned into a neoR containing the lentiviral vector using the Gateway cloning system according to the manufacturer’s instructions. Generation and titre of virus Viral production was performed by co-transfecting neo HA hPar1 vector orneo HA hPar1 7A vector (2 μg) and packaging vectors pCMVΔR8.91 (1.8 μg) and pMD2.VSVG (0.2 μg) into HEK293T cells using 12 μl TransIT LT1 transfection reagent (Mirus Bio LLC) in 100-mm plates. The resulting supernatant was collected after 48 and 72 h. The virus was recovered after ultracentrifugation for 1 h at 42,000 r.p.m. in a Beckman SW28 rotor (Beckman-Coulter, Brea, CA, USA). The resulting pellet was resuspended in medium to reach 100 × the initial viral concentration. Various hPar2 constructs, wt hPar2 , and truncated and deleted hPar2 C-tail constructs, as well as mutants of hPar2 were cloned into lentiviral vectors. Preparation of stable clones MCF7 cells were infected with HA- hPar1 virus or hPar1 -7A virus. This was followed by selection using Geneticin G418 resistance (500 μg ml −1 ) to produce MCF7- hPar1 and MCF7- hPar1-7A stable clones. To obtain MCF7- hPar1- Etk/Bmx and MCF7- hPar1-7A -Etk/Bmx stable clones, infection of Etk/Bmx virus was performed to the above-mentioned clones. Clone efficiency was evaluated using RT–PCR and western blotting. HU stable clones stably expressing hPar2wt and various deletion constructs, as well as mutants, were similarly generated. Mammary gland mouse model Female athymic nude mice aged 6–7 weeks were pre-implanted subcutaneously with pellets containing 1.7 mg β-estradiol (60-day release, Innovative Research of America, Sarasota, FL, USA). Mouse mammary fat pads were then injected with 5 × 10 6 MCF-7 cells stably expressing hPar1 wt , hPar1 wt and Etk/Bmx , hPar1-7A and hPar1-7A and Etk/Bmx constructs, or pcDNA3 control plasmid. Mice were monitored for tumour size by external calibre measurements (length and width) on days 10, 22, 25 and for up to 45 days if tumour burden allowed. Tumour volume ( V ) was calculated by V = L × W 2 × 0.5, where L is length and W is width. At the end of the experiment, mice were killed and tumours were removed, weighed and fixed in formalin for histology. All animal experiments were approved by the animal committee of the Hebrew University (MD-09-11803-2). Histology Tissue samples derived from mouse primary tumours were fixed with 4% formaldehyde in PBS, embedded in paraffin and sectioned (5 μm sections). After deparaffinization and rehydration, the sections were stained with H&E or were subjected to immunohistochemistry using specific antibodies. Immunohistochemistry Paraffin-embedded slides were deparaffinized and incubated in 3% H 2 O 2 . Antigen unmasking was carried out by heating (20 min) in a microwave oven in 10 mM Tris buffer containing 1 mM EDTA. After blocking, slides were incubated with the following primary antibodies: PCNA (sc-56, Santa Cruz Biotechnology, Santa Cruz, CA, USA; dilution 1:200), β-catenin (C-2206, Sigma-Aldrich, St Louis, MO, USA; dilution 1:100) and caspase 3 (9661S, Cell Signaling Technology, Danvers, MA, USA; dilution 1:100) and diluted in CAS-Block (Invitrogen), or with CAS-Block alone, as a control. Appropriate secondary antibodies (Nichirei, Tokyo, Japan; dilution 1:1,000) were then added and the slides were incubated at room temperature for 30 min. Colour was developed using the 3,3′-diaminobenzidine (DAB) (Thermo Scientific, Walham, MA, USA) or the Zymed AEC substrate kit (Zymed Laboratories So., San Francisco, CA, USA), followed by counterstaining with Mayer’s haematoxylin. Controls without addition of primary antibody showed low- or no background staining in all cases. Generation of PAR 2 deletion constructs and mutants PAR 2 deletion mutants were generated with site-directed mutagenesis using QuikChange Lightning Site-Directed Mutagenesis Kit (Agilent Technologies Stratagene, Santa Clara, CA, USA) according to the manufacturer’s instructions. The primers used for insertion of stop codons, invariably along the hPar2 C-tail, and for the generation of mutants R352A and H349A, are shown in Supplementary Table 2 . Membrane solubilization Cells were solubilized in lysis buffer containing 10 mM Tris-HCl (pH 8), 2.5 mM MgCl 2 , 5 mM KCl, 1 mM dithiothreitol, protease inhibitor mixture (1:100), 1 mM phenylmethylsulfonyl fluoride (PMSF) and 1 mM sodium orthovanadate (Sigma-Aldrich) for 30 min at 4 °C. After centrifugation at 12,000 g , the supernatant containing the cytoplasmic fraction was collected and the pellet was resuspended with 1% Triton X-100, 150 mM NaCl and 50 mM Tris acetate (pH 8.2). The supernatants obtained after centrifugation at 12,000 g contained the membrane fraction. This procedure facilitated enrichment of the membrane fraction. Western blot analysis and antibodies Cells were solubilized for 30 min at 4 °C in lysis buffer containing 10 mM Tris-HCl, pH 7.4, 150 mM NaCl, 1 mM EDTA, 1% Triton X-100, a protease inhibitor cocktail (0.3 μM aprotinin, 1 mM PMSF; Sigma-Aldrich and 10 μM leupeptin). After centrifugation at 12,000 g for 20 min at 4 °C, the supernatants were transferred and the protein content was measured. Lysates (50 μg) were loaded on a 10% SDS–PAGE gel followed by transfer to Immobilon-P membrane (EMD Millipore/Merck, Damstadt, Germany). Membranes were blocked and probed with the appropriate antibodies. Anti-HA for IP (1 μg per assay) was obtained from Santa Cruz Biotechnology, and for Western blot (HA.11mAb; 1:500 dilution) from Covance, Berkeley, USA. 1 μg/assay SAM11 antibody (Santa Cruz Biotechnology) was used for IP and a 1:500 dilution was used for Western blot detection of overexpressed hPar2 . Rabbit anti GFP antibody, anti Akt antibody and anti phospho-Akt were obtained from Cell Signaling Technology and used at a dilution of 1:1,000. Mouse anti T7 antibody was obtained from Novagen Madison, WI; and used at a dilution of 1:10,000. Anti β-actin was purchased from Sigma-Aldrich and used at a dilution of 1: 5,000. Uncropped immunbloots and larger blot areas are represented in Supplementary Fig. 12 Immunoprecipitation Protein cell lysates (400 μg) were used for IP analysis. Mouse anti-PAR 2 antibodies were added to the cell lysates. After overnight incubation, protein A-sepharose beads (Sigma-Aldrich) were added to the suspension, which was subsequently rotated at 4°C for 1 h. Elution of the reactive proteins was performed by resuspending the beads in protein sample buffer followed by boiling for 5 min. The supernatant was then resolved on a 10% SDS–polyacrylamide gel and was treated as indicated above for western blot analysis. GST fusion protein Fusion proteins were purified from transformed Esherichia coli (strain BL21) that had been stimulated with isopropyl-β-D-thio-galactopyranoside at a concentration of 0.3 μM. Bacteria were lysed by sonication in solution containing 10 mM Tris-HCl (pH 8.0), 0.5% Nonidet P-40 (NP-40), 100 mM sodium chloride, 20 mM EDTA (pH 8.0) and protease inhibitors. Lysates were then immobilized on glutathione sepharose beads (Pharmacia/GE LifeSciences, Marlborough, MA, USA). Lysates of HEK-293 with and without transfection with T7-Etk/Bmx, colon carcinoma CL1, HCT-116 and HU cells were loaded on these columns. The bound proteins were then washed and sample buffer was added and loaded on SDS–PAGE, followed by immunoblotting with the indicated antibodies and ECL detection. GST- h PAR 2 -C-tail cloning The C-tail fragment of h PAR 2 , containing 52 amino acids from residue 346 (phenylalanine) to residue 397 (tyrosine), was prepared using PCR amplification (using primers containing Eco RI and Bam HI restriction sites (respectively, indicated by underlined letters): 5′-CG GAATTC TTTGTTTCACATGATTTCA-3′ and 5′-CG GGATCC ATAGGAGGTCTTAACAGT-3′). The resulting DNA fragment was further cut with the appropriate restriction enzymes ( Bam HI and Eco RI) and ligated into the pGEX-2T vector. GST- h PAR 2 K378Z-C-tail and GST- h PAR 2 K356Z-C-tail were also prepared using the same technique. The suitability of the constructs was confirmed by dideoxy sequencing followed by SDS–PAGE separation, which indicated that the fusion proteins of the C-tails were adequately prepared. The molecular weights of GST fusion proteins were as follows: 27 kD for GST itself, 32.9 kD for the GST- h PAR 2 -C-tail, 30.7 kD for the GST- h PAR 2 K378Z-C-tail, 28.2 kD for the GST- h PAR 2 K356Z-C-tail, 45 kD for GST-PH-Akt and 80 kD for GST-PH-Vav 3 . GST-PH-Etk/Bmx The PH domain in Etk/Bmx was bound to the GST column as previously described [27] . Briefly, GST fusion proteins and His-T7-tagged proteins were expressed in bacteria and purified by using glutathione sepharose (Pharmacia) or Ni 2+ column (Novagen) as recommended by the manufacturers. The purified GST fusion proteins remained on the glutathione sepharose beads and were then mixed with purified His-T7-tagged PH domain in PBS containing 0.5 mg ml −1 bovine serum albumin. After overnight incubation, the beads were collected and extensively washed with cold PBS. The bound proteins were analysed using SDS–PAGE followed by western blot analysis with anti-T7 antibody. The GST-PH-Akt construct was kindly provided by Dr Brian A. Hemmings (Friedrich Miescher Institute). The GST-PH-Vav 3 construct was kindly provided by Dr Shan Lu (University of Cincinnati College of Medicine). HA-tag wt hPar1 and HA-mutant hPar1- 7A C-tail constructs Mutants were designed for insertion of A at the carboxy terminus of PAR 1 residues 378–384: SSE CQRYVYS ILCCKESS to SSE AAAAAAA ILCC (named hPar1 -7A mutant). For HA-tag wt hPar1 construct PCR primers were designed and added downstream to the ATG start codon. Primers for the HA-tag were as follows: sense: 5′-TACCCATACGATGTTCCAGATTACGCT-3′ and antisense: 5′-AGCGTAATCTGGAACATCTATGGGTA-3′. Replacement of seven residues with Ala (A) at positions 378–384 was performed by synthesis of oligos containing the mutation. Primer sequences were as follows: hPar1 7A mutant: sense: 5′-TCTGAGGCTGCTGCTGCTGCTGCAGCTATCTTA-3′ and antisense: 5′-TAAGATAGCTGCAGCAGCAGCAGCAGCCTCAGA-3′. PCR products were then used as primers on an hPar1 cDNA template to create an extended product of mutations introduced into the full-length sequence. The amplified DNA fragment was digested with Pin AI and Xba I from PAR 1 cDNA and was cloned into pcDNA3- hPar1 plasmid followed by DNA sequencing. Placenta tissue collection and preparation Placental tissues were prepared as previously described [35] . Briefly, the placental tissues were extracted from discarded material provided by patients who voluntarily and legally chose to terminate pregnancy during the first trimester (between 5- and 12-week gestation). Gestational age was determined by the date of the last menstrual period and ultrasound measurement of fetal crown-rump length. All specimens were obtained strictly in adherence with the Hadassah-Hebrew University Institutional Ethics Committee Guidelines (we received informed consent from women who voluntarily and legally chose to terminate pregnancy; Helsinky 0436-13-HMO; serial number 123130). First-trimester villous explants in cultures The preparation and cultivation of villous explants of various first-trimester placentae was performed as described elsewhere [20] , [35] , [36] , [37] . Briefly, placental tissue originating from samples harvested between 10- and 12-week gestation was immediately rinsed in sterile cold PBS and processed within 2 h of collection. Following dissection under the microscope, ∼ 2–5 mg weight specimens were carefully laid on 200 μl of solid reconstituted undiluted Matrigel substrate (Becton Dickinson, Bedford, MA, USA) in 0.4-μm pore-culture Millicell-CM culture dish inserts (pore size 0.4 μm, Millipore Corp, Bedford, MA, USA). Explants were cultured in DMEM/F-12 supplemented with 100 U ml −1 penicillin, 100 μg ml −1 streptomycin and 0.25 μg ml −1 ascorbic acid, pH 7.4. Villous explants were maintained in culture for 3 days. Viability of the explants was assessed by adherence to Matrigel and emerging EVTs breaking from the tips as observed under a phase microscope. After 24 h in culture, explants were treated with thrombin (1 U ml −1 ), TFLLRN (100 μM) and SLIGKV (100 μM), and were transfected or not with wt hPar1, hPar1 7A mutant or with wt hPar2 and mutant hPar2 H349A viral vectors. After 72 h in culture, the Matrigel cast cylinders with the EVTs were detached from the base of the insert cells by fine dissection under the microscope, fixed in 4% paraformaldehyde, embedded in paraffin and further processed for histochemical tissue analysis. Each experiment was carried out in triplicate using samples originating from eight different placental sets. EVT invasion assessment We assessed the H&E-stained serial sections of the EVT. We limited our study to the trophoblasts that penetrated through the Matrigel but remained on the surface of the polycarbonate membrane, that is, within the cast [35] , [36] , [37] . These were visualized on sequential slices of the entire Matrigel cast by haematoxylin staining. Slides were photographed using the digital image capture software and all specimens were evaluated by two authors (S.G.-G. and M.M.). Depth of invasion was assessed for each experiment (disappearance of trophoblast cells on the serial sections). For each set of experimental conditions, the total number of EVT cells was counted and the mean±s.e.m./high power field (HPF) was calculated for five randomly selected microscope fields (magnification × 40) at the deepest common level of invasion. Statistical analysis At the deepest common level of invasion, the total EVT cells at five randomly selected microscope fields were counted, for each experimental condition and the mean±s.e.m./HPF calculated. The data were statistically evaluated using analysis of variance Tukey honest significant difference (HSD) test of multiple comparison showing a P value of 0.0001 within groups. The mean difference is significant at the 0.05 level. How to cite this article: Kancharla, A. et al. PH motifs in PAR 1&2 endow breast cancer growth. Nat. Commun. 6:8853 doi: 10.1038/ncomms9853 (2015).